Enhanced biofuel production through coupled acetic acid and xylose consumption by engineered yeast The anticipation for substituting conventional fossil fuels with cellulosic biofuels is growing in the face of increasing demand for energy and rising concerns of greenhouse gas emissions. However, commercial production of cellulosic biofuel has been hampered by inefficient fermentation of xylose and the toxicity of acetic acid, which constitute substantial portions of cellulosic biomass. Here we use a redox balancing strategy to enable efficient xylose fermentation and simultaneous in situ detoxification of cellulosic feedstocks. By combining a nicotinamide adenine dinucleotide (NADH)-consuming acetate consumption pathway and an NADH-producing xylose utilization pathway, engineered yeast converts cellulosic sugars and toxic levels of acetate together into ethanol under anaerobic conditions. The results demonstrate a breakthrough in making efficient use of carbon compounds in cellulosic biomass and present an innovative strategy for metabolic engineering whereby an undesirable redox state can be exploited to drive desirable metabolic reactions, even improving productivity and yield. Second-generation biofuels produced from renewable lignocellulosic biomass could serve as a promising and sustainable alternative to conventional fossil fuels in the face of growing demand for energy and rising greenhouse gas emissions [1] , [2] , [3] . In contrast to more prevalent feedstocks such as corn and sugarcane for first-generation biofuel production, lignocellulosic biomass derived from agricultural and forestry residues or industrial wastes could mitigate ‘food versus fuel’ concerns [4] . Further, fuels produced from lignocellulosic biomass can replace substantial amounts of petroleum-based fuels [5] . However, incomplete and inefficient conversion of cellulosic sugars present in solubilized plant cell wall carbohydrates (hydrolyzates) into biofuels has hindered commercial-scale processes. One major bottleneck is the economic conversion of hemicellulose, one of the main structural components in lignocellulosic biomass along with cellulose, into biofuels [6] . The sugar D -xylose, derived from hydrolysis of hemicellulose, is the second most abundant sugar in the plant cell wall consisting of up to 35% of the total carbohydrate from lignocellulosic biomass [7] . However, the yeast Saccharomyces cerevisiae, the most widely used microorganism for producing corn and sugarcane ethanol, cannot metabolize xylose. Further, hemicellulose and lignin in the plant cell wall are acetylated [8] , yielding acetic acid as an unavoidable component in cellulosic hydrolyzates with acetic acid concentrations ranging from 1 to 15 g l −1 (refs 8 , 9 ). Acetic acid is toxic to fermenting microorganisms and negatively influences sugar fermentation and biofuel yields [8] , [10] , [11] , [12] . Xylose conversion and acetic acid detoxification are two major problems that must be solved to make cellulosic biofuels economically viable. Although xylose-fermenting yeasts exist in nature, their ethanol production rates and tolerances are inferior to S. cerevisiae [13] . Therefore, metabolic engineering has been used to develop xylose-utilizing S. cerevisiae strains [7] , [14] , [15] by expression of nicotinamide adenine dinucleotide phosphate (NAD(P)H)-linked xylose reductase (XR) and nicotinamide adenine dinucleotide (NAD + )-linked xylitol dehydrogenase (XDH) genes from Scheffersomyces stipitis ; this pathway converts xylose to xylulose [14] , [16] , which can be metabolized via the pentose-phosphate pathway after phosphorylation ( Fig. 1 ). However, this pathway introduces a problematic redox cofactor imbalance because XR can use both NADPH and nicotinamide adenine dinucleotide (NADH), whereas XDH uses NAD + only, leading to high xylitol accumulation and low ethanol yields [17] , [18] , [19] , [20] . Xylitol formation could be reduced by providing sufficient oxygen [21] . However, aeration has a prohibitively high cost and lowers ethanol yield. Despite decades of research, the use of XR and XDH for ethanol production is still not viable because the XR/XDH pathway cannot be operated optimally under anaerobic conditions [7] , [22] . 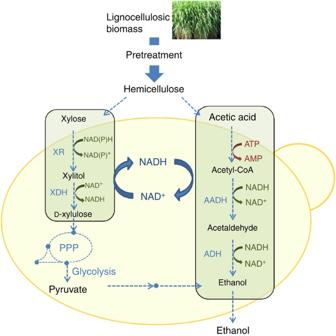Figure 1: EngineeringS. cerevisiaefor co-consumption of xylose and acetic acid. The pathway for xylose metabolism is realized by expressing xylose reductase (XR) and xylitol dehydrogenase (XDH) fromS. stipitis,which produces excess NADH. The pathway to reduce acetic acid is fulfilled with three reactions: (1) EC 6.2.1.1: Acetate+ATP+CoA→Acetyl-CoA+AMP+2Pi, (2) EC 1.2.1.10: Acetyl-CoA+NADH→Acetaldehyde+NAD++CoA and (3) EC 1.1.1.1: Acetaldehyde+NADH→Ethanol+NAD+.S. cerevisiaehas acetyl coenzyme A (acetyl-CoA) synthetase for reaction (1) and alcohol dehydrogenase (ADH) for reaction (3). Expressing acetylating acetaldehyde dehydrogenase (AADH) intoS. cerevisiaeis expected to complete the pathway: Acetate+ATP+2NADH→Ethanol+2NAD+, which can regenerate NAD+from excess NADH in xylose metabolism. Figure 1: Engineering S. cerevisiae for co-consumption of xylose and acetic acid. The pathway for xylose metabolism is realized by expressing xylose reductase (XR) and xylitol dehydrogenase (XDH) from S. stipitis, which produces excess NADH. The pathway to reduce acetic acid is fulfilled with three reactions: (1) EC 6.2.1.1: Acetate+ATP+CoA→Acetyl-CoA+AMP+2Pi, (2) EC 1.2.1.10: Acetyl-CoA+NADH→Acetaldehyde+NAD + +CoA and (3) EC 1.1.1.1: Acetaldehyde+NADH→Ethanol+NAD + . S. cerevisiae has acetyl coenzyme A (acetyl-CoA) synthetase for reaction (1) and alcohol dehydrogenase (ADH) for reaction (3). Expressing acetylating acetaldehyde dehydrogenase (AADH) into S. cerevisiae is expected to complete the pathway: Acetate+ATP+2NADH→Ethanol+2NAD + , which can regenerate NAD + from excess NADH in xylose metabolism. Full size image The acetic acid present in lignocellulosic hydrolyzates is toxic to fermenting microorganisms. In most cases in nature, acetate is metabolized using respiratory metabolism only in the presence of terminal electron acceptors such as oxygen, nitrate, ferric iron and sulphate [23] . Reductive metabolism of acetate occurs during the solventogenic phase by some Clostridium species, where acetate can be converted to ethanol using surplus NADH generated during the acidogenic phase [24] . By contrast to the redox-neutral xylose isomerase (XI) pathway for converting xylose into xylulose [25] , [26] , we reason that the surplus NADH generated from xylose metabolism using the XR/XDH pathway could provide the reducing equivalent for acetate reduction. Conversely, reduction of acetate to ethanol could serve as an electron sink to alleviate the redox cofactor imbalance resulting from xylose fermentation ( Fig. 1 ). Notably, XR-XDH-carrying strains have significantly higher xylose consumption rates, specific ethanol productivity and final ethanol concentration, when compared with otherwise isogenic XI-carrying strains, although XI strains achieve higher ethanol yields [26] . Therefore, here we aim to implement the acetate reduction pathway together with the XR-XDH pathway in S. cerevisiae . This strategy has three major benefits. Firstly, using acetate as a redox sink may increase ethanol yield by increasing carbon flux from both xylose and acetate to ethanol without substantial accumulation of glycerol and xylitol. Secondly, the consumption of acetic acid enables in situ detoxification of lignocellulosic hydrolyzates, lessening their inhibitory effects on the productivity of fermenting microorganisms. Thirdly, co-conversion of cellulosic sugars and the non-carbohydrate component acetic acid to value-added products presents a strategy towards making efficient use of the cellulosic carbon. Anaerobic xylose fermentation by S. cerevisiae strain SR8 Engineered S. cerevisiae strains with the XR/XDH pathway grow extremely slowly when xylose serves as the sole carbon source under anaerobic conditions that are desirable for large-scale industrial fermentation [14] , [27] , [28] . We constructed an efficient xylose-fermenting S. cerevisiae strain SR8 by combining rational and combinatorial approaches [29] . The SR8 strain ferments and grows on xylose under anaerobic conditions as well as oxygen-limited conditions, and the fermentation performance of the SR8 strain was comparable to the best performing engineered S. cerevisiae strains reported previously ( Supplementary Table S1 ). The SR8 strain was tested for its capability to ferment and grow on xylose alone under anaerobic conditions. Around 35 g l −1 xylose was consumed within 60 h ( Supplementary Fig. S1 ). Ethanol was produced with a specific productivity of 0.24 g ethanol per g dry cell weight per hour) to a final concentration of 12.6 g l −1 . Yet, this strain still produced substantial amounts of the reduced by-products xylitol and glycerol ( Supplementary Fig. S1 ), which suggests that the engineered yeast with the heterologous XR/XDH pathway suffers from surplus NADH generated from the XR/XDH reactions. Relationship between NAD + regeneration and product yield As a first step to control the surplus NADH, an external electron acceptor acetoin, which can be reduced to 2R,3R-butanediol (BDO) when coupled with NADH oxidation to NAD + [30] , was introduced into the xylose fermentations. Reduction of acetoin into BDO can be used to illustrate the impact of NAD + regeneration on anaerobic xylose fermentation. Acetoin was reduced to BDO at almost maximum levels according to the stoichiometry ( Supplementary Fig. S2a ). As expected, the supplementation of acetoin decreased the yield of reduced by-products (glycerol and xylitol) from xylose fermentation under anaerobic conditions, allowing for more carbon flux to ethanol ( Supplementary Fig. S2b ). Higher amounts of acetoin reduced to BDO correlated with more ethanol production and less xylitol and glycerol accumulation. These results are consistent with a previous report [30] , and reveal a linear correlation between NAD + regeneration and improvement in xylose fermentation ( Supplementary Methods ). Quantitative evaluation revealed a linear correlation between NAD + regeneration and decrease of the reduced by-product formation ( Supplementary Fig. S2c ). Xylitol yields are also inversely correlated with total NAD + regenerated from acetoin reduction and glycerol production, which confirms that the availability of regenerated NAD + from oxidation of surplus NADH is a crucial factor that limits efficient xylose fermentation under anaerobic conditions [22] , [31] . Expression of acetate reduction pathway Acetoin is not an economically effective additive for improving industrial production of ethanol from lignocellulosic hydrolysates. To explore the potential of using acetate as a redox sink, we evaluated the feasibility of a metabolic pathway for reducing acetate into ethanol by acetyl-CoA through elementary flux mode analysis ( Supplementary Methods ). The elementary flux mode analysis revealed that acetate reduction to ethanol mediated by endogenous acetyl-CoA synthetase (by using ATP to AMP) and heterologously expressed acetylating acetaldehyde dehydrogenase (AADH) (by using NADH as cofactor) could be operational in yeast and serve to alleviate the surplus NADH produced from xylose fermentation ( Supplementary Note 1 ). Acetate reduction was also predicted to increase ethanol yield and reduce by-product yield during xylose fermentation ( Supplementary Fig. S3 ). We therefore introduced the acetate reduction pathway to evaluate whether the presence of acetate could improve xylose fermentation under anaerobic conditions. Five possible AADH enzymes were introduced into the xylose-fermenting S. cerevisiae strain SR8, resulting in different engineered yeast strains as summarized in Table 1 . The selected enzymes can be divided into three types of known AADH functional homologues, including (1) bifunctional proteins that catalyse the reversible conversion of acetyl-CoA to acetaldehyde and the subsequent conversion of acetaldehyde to ethanol (for example, Escherichia coli AdhE, Piromyces sp. E2 AdhE, C. beijerinckii acetaldehyde-CoA dehydrogenase (ALDH)), (2) proteins involved in ethanolamine catabolism (for example, E. coli EutE) and (3) proteins that are part of a bifunctional aldolase–dehydrogenase complex involved in 4-hydroxy-2-ketovalerate catabolism (for example, E. coli MphF). The resulting engineered yeast strains exhibited different capabilities in consuming acetate during the fermentation of 20 g l −1 xylose under anaerobic conditions. Three yeast strains expressing E. coli adhE , E. coli eutE and Piromyces sp. E2 ADHE , consumed acetate from the beginning of fermentation until xylose was depleted. The S-adhE strain had the highest cumulative acetate consumption (0.62 g l −1 ), followed by the S-eutE strain (0.53 g l −1 ) and S-PadhE strain (0.41 g l −1 ; Fig. 2 ). The S-Cbaldh strain expressing C. beijerinckii ALDH consumed only 0.12 g l −1 of acetate at the end of xylose fermentation. The strain S-mphF had no noticeable acetate assimilation, which was similar to the control strain S-nc ( Fig. 2 ). Enzymatic activity assays of the three acetate-assimilating strains confirmed the functional expression of the three AADH genes ( E. coli adhE, eutE or ADHE of Piromyces sp . E2 ; Supplementary Fig. S4 ), whereas the strains S-mphF and S-Cbaldh showed similar results to that of the strain S-nc (data not shown). Table 1 Strains and plasmids used in this study. 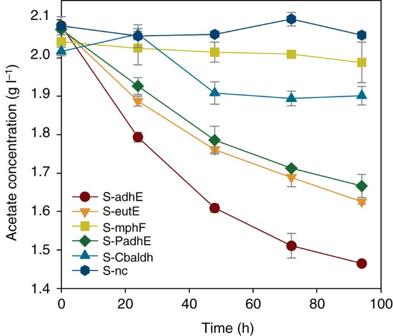Figure 2: Acetate reduction during anaerobic xylose fermentation. Consumption of acetate in xylose fermentation by the yeast strains expressingE. coli adhE(NCBI Gene ID: 945837, strain named S-adhE),E. coli eutE(NCBI Gene ID: 957684, strain named S-eutE),E. coli mphF(NCBI Gene ID: 945008, strain named S-mphF), ADHE from anaerobic fungusPiromycessp. E2(NCBI GenBank: AY282576.1, strain named S-PadhE) and the acetaldehyde-CoA dehydrogenase gene fromC. beijerinckii(NCBI Gene ID: 5291537, strain named S-Cbaldh). S-nc is the control with empty plasmid. Results are the mean of duplicate experiments; error bars represent s.d. and are not visible when smaller than the symbol size. Full size table Figure 2: Acetate reduction during anaerobic xylose fermentation. Consumption of acetate in xylose fermentation by the yeast strains expressing E. coli adhE (NCBI Gene ID: 945837, strain named S-adhE), E. coli eutE (NCBI Gene ID: 957684, strain named S-eutE), E. coli mphF (NCBI Gene ID: 945008, strain named S-mphF), ADHE from anaerobic fungus Piromyces sp . E2 (NCBI GenBank: AY282576.1, strain named S-PadhE) and the acetaldehyde-CoA dehydrogenase gene from C. beijerinckii (NCBI Gene ID: 5291537, strain named S-Cbaldh). S-nc is the control with empty plasmid. Results are the mean of duplicate experiments; error bars represent s.d. and are not visible when smaller than the symbol size. Full size image Under anaerobic conditions, acetate should be metabolized through a reductive pathway rather than through respiration. To confirm the reduction of acetate to ethanol, acetate-2- 13 C was tracked in xylose fermentation experiments using gas chromatography–mass spectrometry (GC–MS) to detect isotopically labelled ethanol. Both isotopically labelled ethanol and its ion fragment were enriched in fermentation samples taken from strains containing the acetate reduction pathway, but not from strains lacking the pathway ( Fig. 3 ; Supplementary Fig S5 ). The abundance ratio of peak 47/46 in samples from fermentation by S-adhE strain was 5.7% ( Fig. 3 ), which is notably higher than that of samples from fermentation by S-nc strain (2.4%) and the control ethanol solution (2.5%) that represents the natural background level of 13 C abundance. These results provide clear evidence that acetate can directly contribute to ethanol production through the introduced reductive pathway. 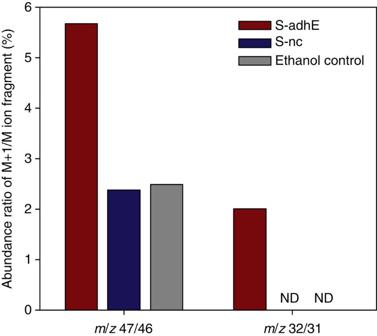Figure 3:13C-ethanol from acetate-2-13C by engineeredS. cerevisiae. Mass spectrum peak abundance ratio ofm/z47 overm/z46 andm/z32 overm/z31 in samples at the end of anaerobic xylose fermentation with acetate-2-13C amendment by strain S-adhE or control strain S-nc, which lacks the gene for acetylating AADH. For ethanol, peak 46 represents the molecular ion and peak 47 represents ethanol with one13C atom; peak 31 represents CH2OH+ion fragment and peak 32 represents13CH2OH+. Ethanol solution was used as the control to show natural abundance of 13C. Each bar represents values from one of two independent replicates, which differed by <5%. Figure 3: 13 C-ethanol from acetate-2- 13 C by engineered S. cerevisiae . Mass spectrum peak abundance ratio of m / z 47 over m / z 46 and m / z 32 over m / z 31 in samples at the end of anaerobic xylose fermentation with acetate-2- 13 C amendment by strain S-adhE or control strain S-nc, which lacks the gene for acetylating AADH. For ethanol, peak 46 represents the molecular ion and peak 47 represents ethanol with one 13 C atom; peak 31 represents CH 2 OH + ion fragment and peak 32 represents 13 CH 2 OH + . Ethanol solution was used as the control to show natural abundance of 13C. Each bar represents values from one of two independent replicates, which differed by <5%. Full size image Effect of acetate reduction on anaerobic xylose fermentation Acetate reduction also improved the efficiency of anaerobic xylose fermentation, increasing both ethanol yield and productivity ( Supplementary Fig. S6a,b ). Overexpression of E. coli adhE substantially increased ethanol yield (0.378±0.002 g per g substrate) by 17% compared with that of the control strain S-nc (0.323±0.001 g per g substrate; Supplementary Fig. S6a ), and overexpressions of E. coli eutE or Piromyces sp . E2 ADHE also enhanced ethanol yields ( Supplementary Fig. S6a ). A linear correlation was observed ( Fig. 4a ); when more acetate was consumed, higher ethanol yields could be achieved. In addition, the S-adhE strain had 21% higher specific ethanol productivity than the S-nc strain ( Supplementary Fig. S6b ). Conversely, accumulation of the reduced by-products (xylitol and glycerol) was greatly reduced ( Supplementary Fig. S6c ). S-adhE strain produced the least amount of glycerol and xylitol among all the strains tested, whereas S-eutE and S-PadhE also had less by-product accumulation than the control strain. The inverse proportional relationship between acetate consumption and reduced by-product yields illustrated in Fig. 4b shows the beneficial effects of the acetate reduction pathway via improved regeneration of NAD + during xylose fermentation. A more detailed comparison of the product yields and NAD + regeneration between the strains S-adhE and S-nc ( Supplementary Table S2 ) also revealed that implementation of the acetate reduction pathway increased the total NAD + generation by nearly 50% while decreasing the need of NAD + generation from glycerol production. 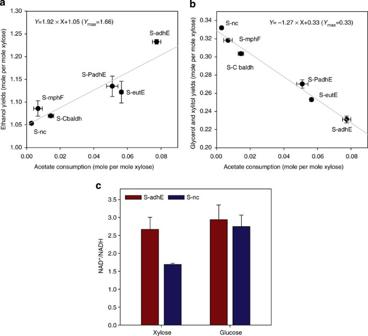Figure 4: Effects of acetate reduction on product yields and redox cofactor balance. (a) Correlation between ethanol yields and acetate consumption inS. cerevisiaestrains. (b) Correlation between accumulation of by-product (glycerol+xylitol) and acetate consumption. Grey lines represent the linear regression curves. (c) Intracellular ratio of NAD+/NADH inS. cerevisiaestrain S-adhE and control strain S-nc in late exponential phase samples in media containing 20 g l−1xylose or glucose and 2 g l−1acetic acid under anaerobic conditions. Results in all the figures are average of biological duplicates, and error bars represent s.d. Figure 4: Effects of acetate reduction on product yields and redox cofactor balance. ( a ) Correlation between ethanol yields and acetate consumption in S. cerevisiae strains. ( b ) Correlation between accumulation of by-product (glycerol+xylitol) and acetate consumption. Grey lines represent the linear regression curves. ( c ) Intracellular ratio of NAD + /NADH in S. cerevisiae strain S-adhE and control strain S-nc in late exponential phase samples in media containing 20 g l −1 xylose or glucose and 2 g l −1 acetic acid under anaerobic conditions. Results in all the figures are average of biological duplicates, and error bars represent s.d. Full size image Fermentation experiments using the best acetate-assimilating strain S-adhE were performed in medium buffered at pH 4.7 (the pKa of acetic acid), where increased concentration of an undissociated form of acetic acid at relatively low pH would increase its toxicity to cells. The strain S-adhE co-consumed acetic acid in anaerobic fermentation of xylose ( Supplementary Fig. S7a ) and had higher ethanol yields ( Supplementary Fig. S7b ). The pH values at the end of fermentation were 5.1 for S-adhE and 4.9 for S-nc. Noticeably, the strain S-adhE grew better ( Supplementary Fig. S7c ) and had faster fermentation rates than the control strain S-nc, which indicates that assimilation and reduction of acetic acid likely alleviates its toxicity. In addition, we tested the fermentation performance of the strain SR7-adhE ( Table 1 ), which has the same genetic background as S-adhE with an intact ALD6 (encoding aldehyde dehydrogenase), under the same experimental condition as that for S-adhE. For the SR7-adhE strain, acetate reduction occurred and helped improve ethanol production ( Supplementary Fig S8 ), which is consistent with the results seen with S-adhE. However, strain SR7-adhE consumed less acetic acid (0.26 g l −1 ) at the end of fermentation of 20 g l −1 xylose compared with S-adhE (0.62 g l −1 ). Moreover, the control strain SR7-nc had a net production of acetic acid ( Supplementary Fig. S8a ). These results indicate that generation of acetate by aldehyde dehydrogenase can compete with acetate assimilation and that ALD6 deletion is beneficial to the strategy. Intracellular NAD + and NADH levels Intracellular concentrations of NAD + and NADH in the S-adhE and S-nc strains in the late exponential growth phase in anaerobic media containing 20 g l −1 xylose or glucose with 2 g l −1 acetic acid were measured. Consistent with the increased ethanol and decreased by-product yields, the ratio of intracellular NAD + to NADH was much higher in strains expressing the acetate reduction pathway during xylose fermentation ( t -test, P =0.0019; Fig. 4c ; Supplementary Table S3 ). In glucose fermentation, where the acetate reduction pathway is not critical for anaerobic fermentation, the ratio of NAD + to NADH was generally high ( Fig. 4c ; Supplementary Table S3 ), which is consistent with the idea that xylose metabolism regenerates NAD + less efficiently than glucose metabolism in S. cerevisiae . Further, the NAD + /NADH ratio of the S-adhE and S-nc strains during glucose fermentation did not show significant differences ( t -test, P =0.422; Fig. 4c ). Taken together, the inverse relationship between acetate consumption and by-product yield ( Fig. 4b ), and measured intracellular concentrations of NAD + and NADH ( Fig. 4c ) provide strong evidence that acetate reduction serves as a viable route for NAD + regeneration during xylose fermentation. Anaerobic fermentation with mixed sugars and acetic acid As a more realistic test of anaerobic co-utilization of xylose and acetate, a simulated fermentation medium mimicking the sugar and toxic acetic acid concentrations of cellulosic hydrolysates (20 g l −1 glucose, 80 g l −1 xylose and 2 g l −1 acetic acid) was used in test fermentations ( Fig. 5 ). Glucose was quickly consumed followed by simultaneous consumption of xylose and acetate within 88 h ( Fig. 5a ). We observed a clear co-consumption of acetate and xylose ( Fig. 5a ), indicating the coupling of the two processes. In contrast, the control strain lacking the acetate reduction pathway did not consume acetate appreciably and exhibited much slower sugar consumption ( Fig. 5b ). Noticeably, the strain containing the acetate reduction pathway grew better ( Fig. 5c ) and produced ethanol faster ( Fig. 5a ), suggesting the beneficial effects of acetic acid reduction. The ethanol yield by S-adhE fermentation (0.414 g per g) was 6% higher than that by the control strain S-nc (0.390 g per g). The acetate reduction pathway resulted in 11% lower by-product yield in S-adhE fermentation relative to the control. The improved ethanol production from co-utilization of xylose and acetate was also demonstrated in synthetic medium and corn stover hydrolysates ( Supplementary Figs S9 and S10 ). In lignocellulosic hydrolysates, reduction of alternative electron acceptors such as furaldehyde compounds might also help improve xylose fermentation [31] , [32] , [33] . However, acetate reduction still occurred in the hydrolysates and improved ethanol yields by strain S-adhE as compared with S-nc, although both strains could conceivably use alternative electron acceptors. 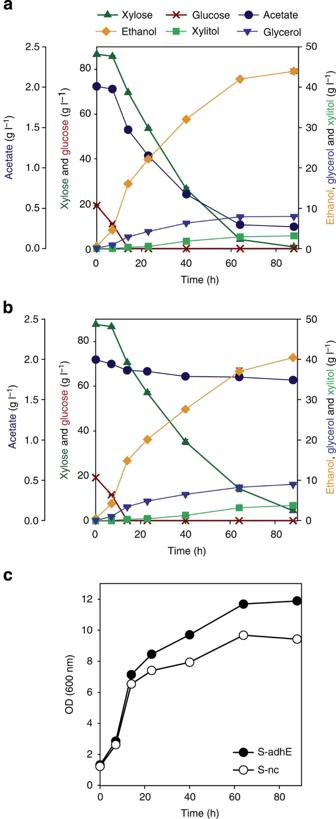Figure 5: Anaerobic fermentation of concentrated mixed sugars. (a) Consumption of xylose, glucose and acetate by S-adhE and production of ethanol. Also shown is the fermentation profile of strain S-nc (b). Results are the mean of duplicate experiments; error bars indicating s.d. are not visible when smaller than the symbol size. (c) Cell growth (OD600) comparison for S-adhE and S-nc. Results are the mean of duplicate experiments; error bars represent s.d. and are not visible when smaller than the symbol size. Figure 5: Anaerobic fermentation of concentrated mixed sugars. ( a ) Consumption of xylose, glucose and acetate by S-adhE and production of ethanol. Also shown is the fermentation profile of strain S-nc ( b ). Results are the mean of duplicate experiments; error bars indicating s.d. are not visible when smaller than the symbol size. ( c ) Cell growth (OD600) comparison for S-adhE and S-nc. Results are the mean of duplicate experiments; error bars represent s.d. and are not visible when smaller than the symbol size. Full size image The use of S. cerevisiae to make ethanol has a long history, but this yeast has not been adapted to use carbon sources such as xylose and acetate derived from plant cell walls. Here we engineered a new pathway not present in nature into yeast to couple xylose fermentation and acetate detoxification under industrially relevant anaerobic conditions. Although the XR/XDH pathway usually generates surplus NADH compared with the alternative redox-neutral XI pathway [34] and results in wasteful by-products, we show that the surplus NADH can be used as an advantage to drive reduction of acetate into ethanol. Meanwhile, the ATP need for activating acetate to acetyl-CoA before AADH reaction may be provided by the co-fermentation of xylose. The strategy is particularly meaningful in that acetic acid, a ubiquitous inhibitor from lignocellulosic hydrolysates, can be co-consumed with cellulosic sugars and thus deliver beneficial effects on sugar fermentation. The acetate reduction pathway implemented here consumes two reducing equivalents (NADH), requiring acetate metabolism to be coupled to reactions that generate NADH to maintain cofactor balance. In contrast to xylose fermentation, glucose fermentation does not generate surplus NADH ( Fig. 4c ), and no acetate reduction occurred when the strain S-adhE was grown in media containing glucose and acetate. A key glycerol production pathway has to be blocked to realize acetate reduction in the presence of glucose, as reported in a previous study where GPD1 and GPD2 were deleted and the E. coli mphF gene was overexpressed [35] . Further, although deletion of GPD1 and GPD2 improve ethanol yield by 13% in fermentation of 20 g l −1 glucose and consumption of about 0.5 g l −1 acetate, deletion of these two genes resulted in compromised cell growth and a substantial decrease in ethanol productivity [35] . The two enzymes Gpd1 and Gpd2 also have crucial roles in osmoregulation and phospholipid biosynthesis [36] . Therefore, deletion of GPD1 and GPD2 for the operation of the acetate reduction pathway would not be a feasible strategy for producing cellulosic biofuels. Whereas the use of E. coli mphF enabled acetate reduction in glucose fermentations in strains lacking GPD1 and GPD2 (ref. 35 ), mphF could not support the acetate reduction pathway in the presence of xylose ( Fig. 2a ). We found the E. coli adhE gene worked best for acetate assimilation and ethanol yield improvement in the xylose-fermenting strains. To our knowledge, this is the first study that demonstrated heterologous expression of E. coli adhE gene in yeast to allow simultaneous fermentation of xylose and acetate prevalent in lignocellulosic hydrolysates under anaerobic conditions. Although the acetate reduction pathway requires ATP for the acetyl-CoA synthase reaction, we observed that the strain S-adhE grew as well as or even better than the control strain S-nc under all the tested conditions ( Fig. 5c ; Supplementary Figs S7c, S9c and S10c ). Particularly, in media with a pH equal to the pKa (4.7) of acetic acid, substantial amounts of undissociated form of acetic acid enters the cells, lowering the intracellular pH and leading to the intracellular accumulation of the acetate anion [37] . As a result, the intracellular pH needs to be recovered by pumping out protons at the expense of ATP hydrolysis, which may negatively influence cell growth. Interestingly, we observed that implementing the acetate reduction pathway resulted in better cell growth ( Supplementary Fig. S7c ). As another mechanism of inhibition by acetic acid is anion accumulation [37] , it is likely that acetate reduction also alleviated acetate anion accumulation inside the cells and reduced its toxicity. Finally, consumption of acetate helped increase pH to a small degree, which might also contribute to the enhanced cell growth and fermentation rates by S-adhE. The present results suggest that ATP supply was not a limiting factor here, that is, the effect of additional ATP consumption by implementing the acetate reduction pathway had a less negative effect on cell growth than the beneficial effect the pathway might bring during anaerobic xylose fermentation. By combining the NADH-producing xylose utilization pathway and NADH-consuming acetate reduction pathway, engineered yeast co-consumed xylose and fermentation inhibitor acetate under anaerobic conditions. Although acetate is converted to ethanol in the present implementation, the yeast strain could be engineered to produce other value-added products or fuels from the co-consumption of xylose and acetate. The results reported in this study demonstrate a breakthrough in making efficient use of carbon compounds in cellulosic biomass, and this strategy will help to make cellulosic ethanol economically feasible. Moreover, the present results demonstrate an innovative metabolic engineering strategy whereby an undesirable redox state of a metabolic pathway can be exploited as a driving force to realize desirable metabolic reactions, even improving productivity and yield. Strains and plasmids The recombinant S. cerevisiae strain SR8 was used in this study for expressing acetate reduction pathway. The strain was constructed previously in our lab [29] through (i) heterologous expression of XYL1 (coding for XR), XYL2 (coding for XDH) and XYL3 (coding for XK) from S. stipitis in S. cerevisiae D452-2 ( MAT α leu2 ura3 his3 and can1 ), and optimization of expression levels of XR, XDH and XK, (ii) laboratory evolution on xylose and (iii) deletion of ALD6 coding for aldehyde dehydrogenase. To introduce an acetylating AADH pathway into the strain SR8, five different genes coding for acetylating AADH were selected, including E. coli adhE (NCBI Gene ID: 945837) , E. coli mphF (NCBI Gene ID: 945008) , E. coli eutE (NCBI Gene ID: 957684), ADHE from anaerobic fungus Piromyces sp . E2 (NCBI GenBank: AY282576.1) and the ALDH gene from C. beijerinckii (NCBI Gene ID: 5291537). The coding regions of the genes were amplified by PCR from E. coli K-12 or C. beijerinckii genomic DNA using primers listed in Table 1 . The sequence of Piromyces sp . E2 ADHE was codon optimized for S. cerevisiae and synthesized by GeneArt . The amplified products were cloned into the pRS425 vector with GPD promoter and CYC terminator. The antibiotic resistance gene KanMX was introduced into the plasmid constructs because the auxotrophic markers were already used in constructing the yeast strain SR8. The plasmid constructs used in this work are summarized in Table 1 . Enzymatic and chemical materials Restriction enzymes, DNA-modifying enzymes and other molecular reagents were obtained from New England Biolabs (Beverly, MA), Promega (Madison, WI), Stratagene (La Jolla, CA) and Roche Biochemical (Indianapolis, IN). The reaction conditions were those recommended by the suppliers. All general chemicals were purchased from Sigma (St. Louis, MO). Primers for both PCR and sequencing were synthesized by Integrated DNA Technologies (Coralville, IA). Yeast transformation Transformation of the plasmid constructs into S. cerevisiae was performed using the yeast EZ-Transformation kit (BIO 101, Vista, CA) and positive yeast transformants were selected on yeast extract-peptone-dextrose (YPD) agar plates supplemented with 200 μg ml −1 of Geneticin G418. The resulting transformants were named as S-adhE, S-mphF, S-eutE, S-PadhE, S-Cbaldh and S-nc (the control with plasmid containing no gene insert). Transformation of expression cassettes containing the selected genes was confirmed by colony PCR using the corresponding primers listed in Supplementary Table S4 . The strains used in this work are summarized in Table 1 . Diagnostic PCR confirmed the successful introduction of the target genes. Medium and culture conditions Yeast strains were routinely cultivated at 30 °C in yeast extract-peptone (YP) medium (10 g l −1 of yeast extract and 20 g l −1 of peptone) containing 20 g l −1 of D -glucose (YPD). E. coli was grown in Luria–Bertani medium at 37 °C, and 50 μg ml −1 of ampicillin was added to the medium when required. To select yeast transformants using the KanMX resistance gene marker, YPD agar plate containing 200 μg ml −1 G418 was used. Pre-culture of yeast strains was cultivated in either YPD media or YPD+G418 media depending on the purpose of different fermentation experiments as below. Anaerobic fermentation experiments Anaerobic batch fermentation experiments were performed at 30 °C in serum bottles sealed with butyl rubber stoppers. For anaerobic xylose fermentation with acetoin as an external electron acceptor, pre-cultured cells in YPD medium were centrifuged and washed twice by sterilized water. The collected cells were inoculated into 20 ml YP medium containing 40 g l −1 xylose or glucose and different concentrations of acetoin (ranging from 5 to 30 g l −1 ). The media were prepared by flushing with nitrogen, which had passed through a heated, reduced copper column to remove traces of oxygen. Initial cell densities were adjusted to around optical density (OD) 600 =1. For anaerobic xylose fermentation with acetate reduction by the engineered yeast strains, pre-cultured cells in YPD+G418 medium were centrifuged and inoculated into 20 ml YP+G418 or synthetic complete (SC)+G418medium containing 20 g l −1 xylose, 40 g l −1 xylose+20 g l −1 glucose or 80 g l −1 xylose+20 g l −1 glucose, and 2 g l −1 acetic acid in serum bottle. For the fermentation experiment to track acetate reduction to ethanol, 2 g l −1 acetate-2- 13 C (Sigma-Aldrich) was used instead of normal acetate. Ergosterol and Tween 80 were added to final concentrations of 0.01 and 0.42 g l −1 , respectively [27] . The anaerobic condition was prepared as described above. For the low pH test, the pH of the YP medium containing 20 g l −1 xylose and 2 g l −1 acetic acid was adjusted to 4.7 buffered by 50 mM potassium phthalate. Initial cell densities were adjusted to around OD 600 =1. All fermentations were performed in duplicate at 30 °C and 100 r.p.m. A similar batch fermentation experiment was also performed with 20 g l −1 glucose in lieu of xylose for comparison. Yeast cell dry weight was determined using a microwave method modified from what was described previously [38] . Briefly, the yeast cell suspension (10 ml) was centrifuged at 4,000 g for 10 min, the pellet was washed twice with distilled water and filtered through a pre-dried and weighed filter. Then, the filter was dried in a microwave oven at 900 W to constant weight. The dry cell weight and OD 600 relationship was determined and was used in metabolic flux calculation. Fermentation of lignocellulosic hydrolysate The corn stover hydrolysate was prepared by National Renewable Energy Laboratory ( http://www.nrel.gov/biomass/pdfs/47764.pdf ). The hydrolysate was mixed with water at 1:1 ratio and centrifuged. The supernatant was collected and filtered. The filtrate was supplemented with concentrated autoclaved YP medium to result in a hydrolysate mixture with 1% yeast extract and 2% peptone. The pH was adjusted to 5.5 using NaOH when needed. The hydrolysate liquid contained about 2.5 g l −1 acetic acid, 18 g l −1 xylose, 2.9 g l −1 glucose and 9.5 g l −1 cellodextrin. Anaerobic fermentation experiments with the strain S-adhE and S-nc in the hydrolysate liquid (amended with 200 μg ml −1 of G418) were set up in serum bottles as described previously. For simultaneous saccharification fermentation, 2% cellulase and 0.4% cellobiase were added into the hydrolysate liquid to enzymatically hydrolyse cellodextrin and cellobiose. All fermentations were performed in duplicate at 30 °C and 100 r.p.m. Enzymatic activity assays Cell extracts from anaerobic xylose-fermenting cultures during exponential phase were prepared by Y-PER Yeast Protein Extraction Reagent (Pierce, Rockford, IL) as described by the supplier, and were used for enzymatic assays of NAD + -dependent acetylating AADH activity. Protein concentrations in cell extract were determined by Thermo Scientific Pierce BCA Protein Assay Kit (Thermo Scientific) as described by the supplier. The enzymatic reaction was initiated by adding 0.6 mM acetyl coenzyme A into the reaction mixture containing 50 mM potassium phosphate buffer (pH 7.5), 0.15 mM NADH and cell extract (total volume 200 μl). The AADH (acetylating) activity was measured by detecting oxidation of NADH from absorbance changes at 340 nm at 30 °C using BioTek’s Synergy HT plate reader (Biotek, Winooski, VT). Analysis was performed for duplicate fermentation experiments, and enzymatic assay was performed in triplicate. Intracellular NAD + /NADH assays Yeast culture samples of strain S-adhE and strain S-nc were withdrawn from anaerobic xylose/glucose fermentation experiments (as described above) during late exponential phase of cell growth. The cells were quenched with cold methanol (−40 °C, 80%), collected by centrifugation, and then washed with cold PBS. The samples were homogenized in NAD(H) extraction buffer and the intracellular NAD + or NADH was extracted and measured using an Enzychrom NAD + /NADH assay kit (Bioassay Systems, Hayward, CA) according to the manufacturer’s instructions. Analytical methods Cell growth was monitored by OD at 600 nm using UV-visible Spectrophotometer (Biomate 5, Thermo, NY). Xylose, glucose, glycerol, xylitol, acetate, ethanol, acetoin and BDO concentrations were determined by HPLC (Agilent Technologies 1200 Series) equipped with a refractive index detector. A Rezex ROA-Organic Acid H+ (8%) column (Phenomenex Inc., Torrance, CA) was used. The column was eluted with 0.005 N H 2 SO 4 as a mobile phase at a flow rate of 0.6 ml min −1 at 50 °C. Samples were taken by sterile syringe and 26G BD needles. Agilent GC/MS system (Agilent Inc, Palo Alto, CA, USA) consisted of a 7,890 gas chromatograph; 5,975 MSD was used to analyse the presence of 13 C-ethanol in samples from fermentation with acetate-2- 13 C amendment. Growth medium after removal of cells was directly injected into GC/MS system. GCy was performed on a 30-m HP-5MS column with 0.25 mm inner diameter and 0.25 μm film thickness (Agilent Technologies) with an injection temperature of 250 °C, the interface set to 250 °C and the ion source adjusted to 230 °C. The nitrogen carrier gas was set at a constant flow rate of 0.8 ml min −1 . The temperature programme was initially 5 min at 40 °C followed by an oven temperature increase of 40 °C min −1 to 280 °C for a final 1 min. The mass spectrometer was operated in positive electron impact mode at 69.9 eV ionization energy in m / z 30–800 scan range. The spectra of all chromatogram peaks were evaluated using the HP Chemstation (Agilent). How to cite this article: Wei, N. et al. Enhanced biofuel production through coupled acetic acid and xylose consumption by engineered yeast. Nat. Commun. 4:2580 doi: 10.1038/ncomms3580 (2013).